Enhanced magnetic Purcell effect in room-temperature masers Recently, the world’s first room-temperature maser was demonstrated. The maser consisted of a sapphire ring housing a crystal of pentacene-doped p -terphenyl, pumped by a pulsed rhodamine-dye laser. Stimulated emission of microwaves was aided by the high quality factor and small magnetic mode volume of the maser cavity yet the peak optical pumping power was 1.4 kW. Here we report dramatic miniaturization and 2 orders of magnitude reduction in optical pumping power for a room-temperature maser by coupling a strontium titanate resonator with the spin-polarized population inversion provided by triplet states in an optically excited pentacene-doped p -terphenyl crystal. We observe maser emission in a thimble-sized resonator using a xenon flash lamp as an optical pump source with peak optical power of 70 W. This is a significant step towards the goal of continuous maser operation. Historically, solid-state masers employing paramagnetic crystals have typically required large static magnetic fields to provide the necessary Zeeman splitting of the electronic spin states in addition to cryogenic cooling to reduce the detrimental effects of lattice vibrations on the lifetime of spin-polarized population inversions [1] , [2] . Efforts to avoid either cryogenic cooling or high magnetic fields have met with limited success. A zero magnetic field solid-state maser [3] using a high quality factor ( Q ) whispering-gallery mode in a single crystal of sapphire with trace paramagnetic Fe 3+ impurities was demonstrated a decade ago, but required cryogenic cooling to liquid helium temperature. The prospect of realizing a room-temperature maser using population inversions within photo-excited triplet-state sublevels in organic paramagnetic molecules was first proposed by Blank [4] , [5] , [6] for a device operating in high magnetic fields. Although maser oscillation was not observed in the reported device, this work paved the way for the recent discovery of maser operation at room temperature and zero magnetic field [7] , which promises a new generation of miniaturized ultra-low-noise high-gain maser amplifiers and oscillators without the incumbent refrigeration and electromagnet infrastructure. Due to their compactness and simplicity, these devices could find application in research areas that rely on detection of weak microwave signals such as structural biology, space science and exploration, communications, quantum information processing and spectroscopy. Stimulated microwave emission at a frequency of 1.45 GHz was observed in a high Q -factor single-crystal sapphire ring housing a single crystal of pentacene-doped p -terphenyl. The pentacene molecules were optically excited from the S 0 singlet ground state into S 1 singlet states by a 350 μs duration pulsed rhodamine-dye laser with wavelength near 590 nm and peak optical power 1.4 kW (see Fig. 1 ). Electrons in the S 1 state rapidly undergo spin-orbit coupling mediated intersystem crossing into the T 2 triplet state with a spin-selective population of the X, Y and Z sublevels in the experimentally determined ratio of 0.76:0.16:0.08 (refs 8 , 9 ). Electrons in the T 2 triplet-state sublevels subsequently relax non-radiatively down into the T 1 triplet state while preserving their spin polarization and resulting in a population inversion between the upper X and lower Z triplet sublevels. Spin-lattice relaxation processes can also occur between the triplet sublevels which eventually decay non-radiatively back to the ground state thus completing the cycle. At zero magnetic field, the frequency splitting between the X and Z triplet sublevels in pentacene-doped p -terphenyl is ~1.45 GHz, so if the spin-polarized paramagnetic molecules are situated within a suitable microwave resonator tuned to this frequency stimulated emission of microwaves due to transitions from the X to Z sublevels may result in amplification of the microwave photons present in the maser resonator if the rate of stimulated microwave emission is greater than the rate of decay due to losses in the cavity. 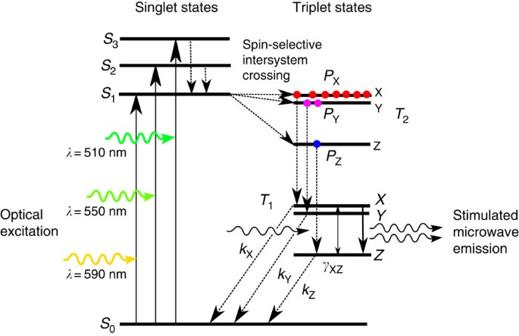Figure 1: Maser process in pentacene. Jablonski diagram showing electronic state cycle responsible for generating population-inverted spin-polarized triplet-state sublevels in pentacene:p-terphenyl. Optical excitation of pentacene molecules from the ground state to the singlet states,S0→S1,S2,S3, followed by spin-orbit coupling mediated spin-selective intersystem crossing from the excited singlet states into theT2triplet manifold. TheT2triplet states decay non-radiatively down to theT1triplet state while preserving the spin-polarized populations. Spin-lattice relaxation can occur between the triplet sublevels with rateγXZ. The triplet sublevels ultimately decay back to theS0ground state with rateskX,Y,Z, thus completing a cycle. X→Z transitions due to stimulated emission lead to amplification of the microwave phonons in the maser cavity. Singlet excitation wavelengths were taken from optical extinction data21. Figure 1: Maser process in pentacene. Jablonski diagram showing electronic state cycle responsible for generating population-inverted spin-polarized triplet-state sublevels in pentacene: p -terphenyl. Optical excitation of pentacene molecules from the ground state to the singlet states, S 0 → S 1 , S 2 , S 3 , followed by spin-orbit coupling mediated spin-selective intersystem crossing from the excited singlet states into the T 2 triplet manifold. The T 2 triplet states decay non-radiatively down to the T 1 triplet state while preserving the spin-polarized populations. Spin-lattice relaxation can occur between the triplet sublevels with rate γ XZ . The triplet sublevels ultimately decay back to the S 0 ground state with rates k X,Y,Z , thus completing a cycle. X→Z transitions due to stimulated emission lead to amplification of the microwave phonons in the maser cavity. Singlet excitation wavelengths were taken from optical extinction data [21] . Full size image The sapphire-based maser operated in burst mode under pulsed optical illumination yet continuous maser operation is essential for a practically usable device. The threshold optical pump power (in pulsed mode) of the original device was estimated to be 230 W and although yellow lasers with such continuous-wave (CW) power output are not currently available, green single-mode fibre lasers are available that could provide the necessary power but they are large, complex and expensive. It seems that the room-temperature maser has replaced the system overhead of cryogenic operation with that of a high-power CW laser with its associated cooling systems and power supplies. However, since almost all the optical power absorbed by the pentacene molecules is transferred into heat, this places an enormous heat load burden on the gain medium, which has a low melting point of 213 °C. One way of relieving the burden of the heat load would be to find superior material systems that provide the necessary microwave paramagnetic gain while reducing heat dissipation. This is the subject of ongoing research in the field. In the meantime, it would also be advantageous to be able to realize room-temperature masers that can operate with reduced optical pumping power requirements. Here we describe a means to dramatically reduce the optical pumping requirement of a room-temperature Earth’s field maser by using a very high permittivity incipient ferroelectric. Two orders of magnitude reduction in the magnetic mode volume and a high Q -factor results in a miniaturized maser that can be optically pumped with a xenon flash lamp delivering peak optical power of 70 W. The estimated optical pump power threshold of this maser is 2 W. Optimizing the magnetic Purcell factor For a maser based on organic paramagnetic triplet systems, the resonators in which they are placed must meet specific criteria for maser threshold conditions to be met. Stimulated transition rates between the triplet sublevels in a molecule such as pentacene are proportional to the magnetic energy density μ 0 | H | 2 and spin–spin relaxation time ( T 2 ). The magnetic energy density can be shown to be inversely proportional to the magnetic mode volume ( V m ), a measure of the physical extent of the resonant mode. The fate of the microwave photons produced by stimulated emission is dictated by their lifetime, which is dependent on the resonator Q -factor. Higher Q -factors mean fewer microwave photons are absorbed by the dielectric and metallic materials from which the resonator is constructed. The ratio of Q -factor and magnetic mode volume was found by Purcell [10] , to provide an explanation for the enhanced spontaneous emission observed in radio-frequency magnetic resonance experiments. The Purcell effect enhances spontaneous and stimulated emission processes and is related to the local electromagnetic density-of-states. The population dynamics of microwave photons and spin-polarized triplet sublevels within a maser can be modelled using coupled differential equations that govern the rate of change in the population of states. For steady-state conditions, a threshold equation for the optical power required to sustain maser oscillation can be derived for a simple two-level system (see Methods): where λ is the optical pump wavelength, κ the optical coupling efficiency, η the intersystem crossing yield, γ the spin-lattice relaxation rate between the X and Z sublevels, P X and P Z the population ratios of the X and Z triplet-state sublevels (0.76 and 0.08, respectively) and k X , k Z their decay rates back to the ground state S 0 . V m is the magnetic mode volume, Q the cavity quality factor and T 2 the spin–spin relaxation time for the X–Z transition. The optical power threshold is inversely proportional to the magnetic Purcell factor: P optical ∝ V m / Q ∝ 1/ F m . The magnetic Purcell factor itself can be optimized by increasing the Q -factor and minimizing the magnetic mode volume V m . Improvement of the Q -factor for a single-crystal sapphire-based resonator by at least an order of magnitude has been reported for a Bragg reflector resonator [11] , however, such resonators have larger mode volumes and are difficult to construct in practice. Alternatively, miniaturizing the maser resonator using high permittivity dielectric materials should reduce the mode volume since it scales as , where ε r is the relative permittivity. This approach has been reported in the field of electron spin resonance spectroscopy [12] , where a potassium tantalate single crystal was successfully used to enhance the signal. Incipient ferroelectrics are very interesting dielectric materials, exhibiting the highest relative permittivities of any non-piezoelectric dielectric. They are classed as incipient (almost) ferroelectrics since their relative permittivity increases dramatically as temperature decreases, suggesting that a ferroelectric phase transition is imminent. However, the phase transition temperature for incipient ferroelectrics is negative and so is not observed. In the case of quantum incipient ferroelectrics, the phase transition temperature is slightly positive but suppressed by zero-point quantum fluctuations. Their very high relative permittivity allows for substantial miniaturization of microwave resonators although their inherent high temperature coefficient of permittivity has excluded them from practical use. Indeed, the first demonstration of a dielectric resonator was constructed from single-crystal rutile but was deemed impractical due to its large temperature coefficient of permittivity [13] . A literature search was conducted to identify dielectric and incipient ferroelectric single crystals that had high relative electrical permittivity and low dielectric loss. Single crystals were chosen since their transparency permits optical excitation of the pentacene: p -terphenyl maser crystal. The candidate materials in addition to sapphire (Al 2 O 3 ) were the incipient ferroelectrics rutile titanium dioxide (TiO 2 ), potassium tantalate (KTaO 3 ) and strontium titanate (SrTiO 3 (STO)) [14] , [15] . Maser resonators incorporating these materials were modelled and their dimensions were optimized to yield maximal Purcell enhancement factors for the TE 01 δ mode resonant at the X↔Z zero-field-splitting frequency near 1.45 GHz. The TE 01 δ mode is advantageous due to its cylindrical symmetry, high quality factor and magnetic field anti-node along its axis. The microwave magnetic field distribution in a TE 01 δ mode resonator resembles a dipole with very strong axial magnetic field strength along the cylindrical axis. The results in Table 1 interestingly show that the magnetic Purcell factor enhancement for a STO maser resonator is over an order of magnitude greater than a sapphire maser resonator. Despite dielectric losses being high in incipient ferroelectrics such as STO, their very high relative permittivities mean that almost all electric and magnetic energy is contained within them when they form dielectric resonators, thus reducing ohmic losses in the metallic cavity walls to negligible levels. Table 1 Purcell factors of candidate masers. Full size table Experimental STO maser performance A maser was constructed from a polished hollow cylinder of STO single crystal (SurfaceNet GmbH) grown by the flame fusion method. The STO cylinder enclosed a pentacene-doped p -terphenyl single crystal (grown in-house) within its bore as shown in Fig. 2 and aligned so that the molecular y -axes of the pentacene molecules had components along the cylindrical axis of the resonator, the same direction as the microwave magnetic field. This was done so that transitions between the X↔Z sublevels could be induced. The nested crystals were housed within a cylindrical copper cavity into which a microwave port (loop on the end of a coaxial cable) was introduced to couple out microwave power generated by stimulated emission. The resonant frequency of the maser could be manually tuned around the X↔Z zero-field transition frequency near 1.45 GHz. The maser output power coupling coefficient was measured using a second microwave port that was very weakly coupled to the maser cavity, allowing a two-port transmission measurement to yield the coupling coefficient of the weakly coupled port (−35 dB). The measured loaded Q -factor of the maser resonator including pentacene: p -terphenyl crystal without optical illumination was 8,900. A poly(methyl methacrylate) (PMMA) light pipe was bonded to the side of the STO resonator and protruded through an aperture in the cavity wall. Broadband optical pulses emitted from a xenon flash lamp (Perkin Elmer MVS 7010) at a repetition rate of 10 Hz were filtered to provide a spectrum in the visible range (450–650 nm) and focussed onto the light pipe which guided them into the cavity and onto the STO/pentacene: p -terphenyl resonator. Microwave power from the coupling port was amplified by a low-noise amplifier (22 dB gain) and fed into a microwave crystal detector (HP Agilent 420A) whose output voltage was recorded by a digital storage oscilloscope (Tektronix TBS 1022). The oscilloscope was triggered by a photodiode that was also used to measure the temporal power profile of the optical pulse emitted at the end of the light pipe near the maser resonator. Based on integrated-sphere measurements of the resonator, it was estimated that the peak optical power absorbed per pulse by the pentacene: p -terphenyl crystal was ~40 W with half-power pulse widths of ~10 μs. On illuminating the maser crystal with an optical pulse from the xenon flash tube, a strong maser burst of microwave power was observed ~20 μs after the onset of the optical pulse with a peak power of 6 μW (−22.2 dBm). The maser burst had a half-power temporal width of ~3 μs and on integration yielded an energy of 2.5 μJ, which corresponds to 2.6 × 10 13 transitions between the X↔Z triplet sublevels accompanied by stimulated emission of microwave photons. Recorded time-domain optical pump and maser output power traces are shown in Fig. 3 along with a two-level rate equation model prediction of the maser output power which agrees well. The experiment was repeated for different resonant frequencies by manually tuning the maser cavity and recording the peak maser output power. The maser produced the strongest signal at 1.4493 GHz as shown in Fig. 4 , which is assumed to be the actual X↔Z zero-field-splitting frequency for the pentacene: p -terphenyl crystal. The width of the frequency response of the maser (~900 kHz) is consistent with reported measurements [16] . 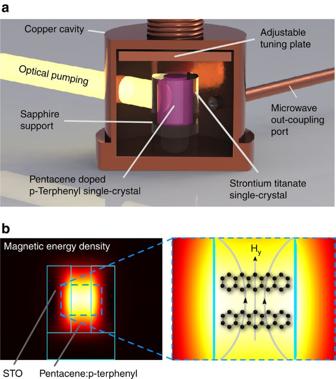Figure 2: Strontium titanate maser construction. (a) Rendered image of strontium titanate (SrTiO3) maser. (b) Plot of magnetic energy-density distribution in the cross-section through maser displaying high concentration within the pentacene:p-terphenyl gain medium. The microwave magnetic field in the TE01δmode behaves like a magnetic dipole and induces X↔Z transitions in the pentacene triplet-state sublevels by having a magnetic field component along the moleculary-axes. Figure 2: Strontium titanate maser construction. ( a ) Rendered image of strontium titanate (SrTiO 3 ) maser. ( b ) Plot of magnetic energy-density distribution in the cross-section through maser displaying high concentration within the pentacene: p -terphenyl gain medium. The microwave magnetic field in the TE 01 δ mode behaves like a magnetic dipole and induces X↔Z transitions in the pentacene triplet-state sublevels by having a magnetic field component along the molecular y -axes. 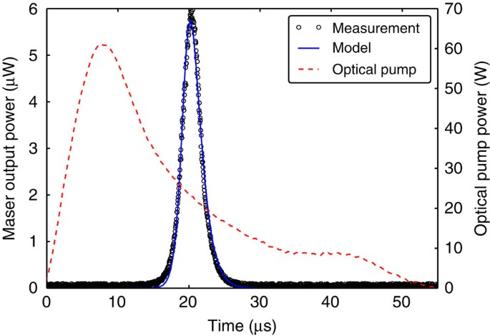Figure 3: Temporal response of maser output power. Measured and modelled microwave burst from strontium titanate/pentacene:p-terphenyl maser excited by xenon flash lamp. Full size image Figure 3: Temporal response of maser output power. Measured and modelled microwave burst from strontium titanate/pentacene: p -terphenyl maser excited by xenon flash lamp. 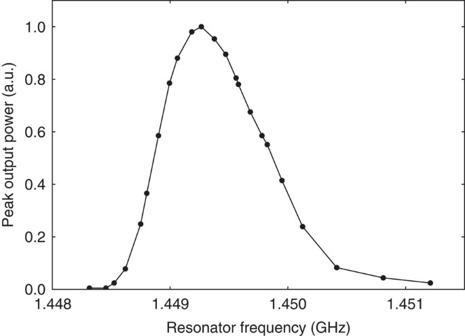Figure 4: Frequency response of STO maser. The peak output power for different resonant frequencies of the TE01δmode, measured on illuminating the pentacene:p-terphenyl crystal within the strontium titanate resonator with a xenon flash lamp. The microwave power was coupled into an low-noise amplifier and detector and measured using a digital storage oscilloscope. The maximum peak power was observed at 1.4493 GHz. Full size image Figure 4: Frequency response of STO maser. The peak output power for different resonant frequencies of the TE 01 δ mode, measured on illuminating the pentacene: p -terphenyl crystal within the strontium titanate resonator with a xenon flash lamp. The microwave power was coupled into an low-noise amplifier and detector and measured using a digital storage oscilloscope. The maximum peak power was observed at 1.4493 GHz. Full size image The time delay between the peak of the optical pulse and the microwave maser emission is due to the finite number of pentacene molecules in the gain medium and the Q -factor of the resonator. Growth in the microwave photon population within the maser mode (amplification) occurs when the rate of stimulated microwave emission exceeds the decay rate due to the losses within the resonator. The population inversion between the X and Z triplet sublevels is depleted until the peak of the maser burst is reached, where the rate of microwave photon production balances the rate of decay due to losses. Although the observed maser bursts only have a peak power of a few microwatts, they are the result of maser amplification of the number of thermal photons present in the cavity from a few thousand to over 10 13 . The total loss of the maser is given by the reciprocal of the loaded quality factor , where Q 0 is the unloaded quality factor of the maser resonator without optical illumination, Q e is the external quality factor due to coupling losses and Q m is the maser gain medium quality factor. The maser medium quality factor Q m can be calculated during simulation, , where U is the energy stored in the maser mode and P m is the stimulated emission power. From simulation, the average gain medium quality factor Q m over the duration of the maser emission was calculated to be 4,500. If the maser medium gain, , is greater than the intrinsic cavity and coupling losses, , then the maser is configured as an oscillator and so the mode energy will grow until saturation or depletion of the inverted population. If the medium gain is greater than the intrinsic cavity losses but less than the total losses, , then the maser is configured as an amplifier with a bandwidth For a bandwidth of 1 MHz, which is approximately the width of the frequency response of maser emission as shown in Fig. 4 , the external quality factor is required to be Q e =1,260. If the gain medium quality factor Q m could be sustained continuously, then the power gain of such a maser when configured as an amplifier could be calculated as [2] : In this case the maser amplifier gain would be 2.7 dB, which although low could be improved by increasing the level of optical pumping power or reducing the bandwidth of the amplifier. For example, reducing the bandwidth to 0.1 MHz would yield a power gain of 12.1 dB. Towards the goal of room-temperature masers being used as high-gain low-noise amplifiers in exciting and possibly new areas of research, here we have demonstrated a considerable step towards the practical realization of such a maser, by reducing the physical volume and optical pumping requirements by almost 2 orders of magnitude. The next step will be to achieve continuous maser operation and explore new organic molecular systems that could provide spin-polarized population-inverted triplet states with possibly more favourable characteristics. Pentacene: p -terphenyl crystal growth Commercially available pentacene powder (TCI Europe NV) was vacuum purified and p -terphenyl commercial powder (Alfa Aesar, 99+%, AL4833) was zone refined. About 0.006% mol per mol pentacene in p -terphenyl powder was prepared and sealed in a 3-mm inner diameter surface modified quartz ampoule with vacuum level of ~10 −3 mbar. A sharp tip was made at one end of the ampoule for self-seeding. The wall surfaces of the ampoule were decorated with 1H,1H,2H,2H-perfluorodecyltrichlorosilane and cleaned thoroughly using solvents (acetone, anhydrous isooctane, isopropanol and distilled water) in an ultrasonic bath. A zone melting technique was used to grow the pentacene-doped p -terphenyl crystal. An in-house furnace’s temperature was controlled with a Eurotherm 3216 temperature controller and TE10A power controller to conduct the zone melting process at an elevated temperature of 200 °C. The melt zone temperature was set at 230 °C. The ampoule was lowered through the furnace at a rate of ~1 mm h −1 using a gear motor. Thereafter, the furnace was cooled down at 1 °C h −1 to room temperature and the ingot retrieved. The zone melting process swept pentacene guest molecules with the melt zone up to the top of the p -terphenyl ingot, leaving that region the most concentrated with pentacene. The top of the ingot with the highest pentacene concentration (determined from the most intense pink colour in the ingot) was selected for the experiments. Due to crystal growth habit, the triclinic c -plane exists along the ampoule long axis. Maser resonator design The maser resonators were modelled using a quasi-analytical radial mode-matching technique [17] . For a given dielectric (Al 2 O 3 , TiO 2 , KTaO 3 or STO) the geometries of the resonators were optimized to yield an optimal magnetic Purcell factor, given by F m =(4 π /3 λ 3 ) Q / V m , where Q is the unloaded quality factor and V m the magnetic mode volume for the fundamental TE 01 δ mode. The unloaded Q -factor is the reciprocal of the sum of the losses within the cavity, such as ohmic losses in cavity walls and dielectric losses within the dielectric resonator and pentacene-doped gain medium. The loss tangent of pentacene-doped p -terphenyl was measured using a dielectric resonator technique and found to be very low (tan δ ~10 −5 ). A low electric filling factor (proportion of electric energy) of the gain medium (<1%) implies that the dielectric losses within the gain medium are almost negligible, confirming that the TE 01 δ mode is an excellent choice for this application. The magnetic mode volume, V m , was calculated as the ratio of the stored magnetic energy within the cavity, μ 0 ∫ V | H ( r )| 2 d V , to the maximum magnetic energy density, μ 0 | H ( r )| 2 . Optimization of the resonator Purcell factors was accomplished using the Nelder–Mead simplex algorithm [18] . Maser population dynamics The triplet-state sublevels X, Y and Z are populated by optical excitation of electrons from the ground state into excited singlet states, which then undergo spin-selective intersystem crossing into the T 2 triplet state with population ratio 0.76:0.16:0.08 for X:Y:Z [8] , [9] . The maser mode at frequency ω is supported by a microwave cavity resonator. Without excitation and in thermal equilibrium with its surroundings, the cavity has a thermal population of ambient microwave photons with a mean photon number given by the Bose–Einstein occupation functions for bosons, . The microwave photon number for the masing cavity mode is then given , where q ′ represents the excess microwave photon number above the thermal level produced by stimulated emission. Spontaneous emission processes were not considered since they are negligible compared with stimulated processes at microwave frequencies. The cavity mode resonant frequency coincides with the splitting between the X and Z triplet manifold sublevels. The optical (pumping) photon power (photon flux) as a function of time is give by p ( t ), the optical coupling efficiency κ from the light pipe into the pentacene: p -terphenyl was estimated to be 50% and the intersystem crossing yield from the excited singlet to the triplet state ( S 1 → T 2 ), η ISC is taken to be 62.5% at room temperature [19] . The rate equations governing the number of cavity photons and electrons in the ground state and triplet sublevels can be written: where T is the triplet population (sum of all X, Y and Z triplet sublevel populations); n 0 is the population of pentacene molecules in the ground state (total available pentacene molecules N ); n X , n Y and n Z are the populations of the X, Y and Z triplet sublevels; P X , P Y and P Z are the triplet sublevel population ratios ( P X + P Y + P Z =1); γ XZ is the spin-lattice relaxation rate between the X and Z sublevels and k X , k Y and k Z are the sublevel non-radiative decay rates back to the ground state. B is the Einstein coefficient for the transition rate of stimulated emission or absorption; q is the microwave photon population of the maser mode; Δ ω is the linewidth of the cavity mode, which is calculated from the loaded Q -factor, Δ ω = ω / Q L . Values for the spin-lattice relaxation rate, γ XZ , and triplet sublevel decay rates were taken from the literature [8] . The microwave photon power coupled out of the cavity at any time is given by P ( t )= q ( t )Δ ωk /(1+ k ), where k is the coupling coefficient of the microwave out-coupling port. The initial number of molecules in the S 0 ground state, n 0 , is equal to the number of pentacene molecules N . Integration of the coupled differential rate equations used a standard solver for systems of coupled partial differential equations. The Einstein coefficient B was calculated from the the magnetic mode volume V m , the spin–spin relaxation time T 2 was taken from ref. 20 and took into account the two different pentacene molecule orientations in the non-equivalent substitution sites in p -terphenyl at room temperature. A steady-state optical pump power threshold equation can be derived by disregarding the Y sublevel and setting the rate of change of cavity photons to zero, leading to: where λ and κ are the wavelength and coupling efficiency of the optical pump source, respectively, V m is the magnetic mode volume and Q is the quality factor. How to cite this article : Breeze, J. et al . Enhanced magnetic Purcell effect in room-temperature masers. Nat. Commun. 6:6215 doi: 10.1038/ncomms7215 (2015).